Iron-based cathode catalyst with enhanced power density in polymer electrolyte membrane fuel cells H 2 -air polymer-electrolyte-membrane fuel cells are electrochemical power generators with potential vehicle propulsion applications. To help reduce their cost and encourage widespread use, research has focused on replacing the expensive Pt-based electrocatalysts in polymer-electrolyte-membrane fuel cells with a lower-cost alternative. Fe-based cathode catalysts are promising contenders, but their power density has been low compared with Pt-based cathodes, largely due to poor mass-transport properties. Here we report an iron-acetate/phenanthroline/zeolitic-imidazolate-framework-derived electrocatalyst with increased volumetric activity and enhanced mass-transport properties. The zeolitic-imidazolate-framework serves as a microporous host for phenanthroline and ferrous acetate to form a catalyst precursor that is subsequently heat treated. A cathode made with the best electrocatalyst from this work, tested in H 2 -O 2, has a power density of 0.75 W cm −2 at 0.6 V, a meaningful voltage for polymer-electrolyte-membrane fuel cells operation, comparable with that of a commercial Pt-based cathode tested under identical conditions. With advantages over the combustion engine including higher fuel efficiency and zero point-of-use emission, combined with those over batteries such as longer operating time and quick refuelling, the H 2 -air polymer-electrolyte-membrane fuel cell (PEMFC) has earned a growing share of the market for material handling vehicle propulsion and backup power systems [1] . However, demonstration fleets and prototypes aside, automotive propulsion still remains an elusive application with numerous challenges [2] , [3] , [4] . The high cost of the PEMFC compared with the gasoline engine, in large part due to the expensive platinum-based catalysts, is a key reason [2] , [3] , [4] . Currently, electrocatalysts account for nearly half of the fuel cell stack cost [5] . Unlike for most components in a PEM FC, economies of scale has little effect on the cost of platinum-based electrocatalysts, because platinum makes up the vast majority of today's catalyst cost [5] . Furthermore, market forces and the highly disproportionate geographical distribution of platinum supply, that is, 90% from South Africa and Russia alone [6] , make the stability and predictability of platinum price nontrivial. Platinum nanoparticles supported on high surface area carbon black is the current practical catalyst technology of choice for H 2 -air PEMFCs [7] , [8] . Meanwhile, several new types of platinum-based electrocatalysts with improved catalytic activity and/or durability have emerged, but are still in development [9] , [10] , [11] , [12] , [13] , [14] . Because the oxygen reduction reaction (ORR) is much slower than the hydrogen oxidation reaction at the anode, the majority of the platinum resides at the cathode. Hence, many of the current research efforts are aimed at producing novel Pt-based catalysts with improved ORR activity [9] , [10] , [11] , [12] , [13] , [14] . Eliminating platinum altogether from cathode catalysts is obviously preferred but has been challenging because of the limited number of catalyst candidates (non-precious metal-based and metal-free) with decent prospects for high ORR activity and durability in acidic medium [15] . Research on Metal/Nitrogen/Carbon-catalysts (M/N/C-) with Co as the metal ion started in 1964 with Jasinski's discovery that a Co-phthalocyanine catalyses the ORR [16] . Catalysts based on Fe as the metal ion later emerged [17] , [18] . The latter was inspired by its similarity to the Fe-heme-copper active centre found in cytochrome c oxidase: an enzyme that catalyses oxygen reduction in both prokaryotes and mitochondria [19] , [20] , [21] , [22] . Today, M/N/C-catalysts obtained from the pyrolysis of elemental precursors and where the metal is either Fe and/or Co are the most promising non-platinum-group-metal (non-PGM) catalysts for the ORR in PEMFCs [10] , [23] . However, to replace platinum-based catalysts, non-PGM catalysts for ORR must still meet the following three criteria: a volumetric activity ≥1/10 that of Pt-based catalysts, excellent mass-transport properties, and high durability. The first two criteria are essential for achieving high power density. Although poor volumetric activity had been a major challenge for M/N/C-catalysts since their discovery, recent breakthroughs have increased their activity to about 1/10 that of Pt-based catalysts [23] , [24] , [25] , [26] , [27] . This level is sufficient for practical applications, [28] , [29] because M/N/C-catalyst loadings of 1–5 mg cm −2 are technically and economically feasible, whereas typical platinum loadings at the cathode are only 0.1–0.4 mg cm −2 to restrain cost [28] , [30] . However, to date, these thicker M/N/C-catalyst cathodes have not yet shown sufficient power density because of poor mass-transport properties intrinsic to the catalyst. For evaluating power density, a fuel cell voltage of 0.6 V is meaningful, because it allows for an acceptable balance between energy efficiency and power density for well-performing catalysts. The highest power densities at 0.6 V reported before this work in H 2 -O 2 PEMFC comprising M/N/C-based cathodes have been 0.38 W cm −2 (ref. 27 ), 0.37 W cm −2 (ref. 26 ), 0.32 W cm −2 (ref. 24 ) and 0.27 W cm −2 (ref. 25 ) with 1.8, 1, 1 and 2 bar back-pressures, respectively. This is significantly lower than the typical value of ca. 1–1.2 W cm −2 attained by a Pt-based cathode with a loading of 0.3 mg Pt cm −2 tested under identical operating conditions. The challenge of achieving a comparable power density with M/N/C-based cathodes at 0.6 V has been especially difficult because, for M/N/C-catalysts, high microporosity is required to obtain high catalytic activity [31] , [32] whereas high meso- or macroporosity has been commonly viewed as a requirement for efficient transport of ORR-related species (O 2 , protons and H 2 O) in the catalyst layer [33] , [34] . In this work, we explore the use of a metal-organic-framework as the host for Fe and N precursors; iron(II) acetate and 1,10-phenanthroline, respectively. The metal-organic-framework (MOF) used in this study is a Zn(II) zeolitic imidazolate framework (ZIF): ZIF-8 (refs 35 , 36 ) (ZnN 4 C 8 H 12 , Basolite Z1200 from BASF). It has a high Brunauer-Emmett-Teller (BET) surface area (upto 1,800 m 2 g −1 , almost entirely microporous), an electrically insulating character before high-temperature treatment and a decomposition temperature of about 500 °C (ref. 35 ). This particular MOF is selected for its high nitrogen content and its high microporous surface area, the two factors that are critical for the ORR activity of Fe/N/C-catalysts [23] , [24] , [31] , [32] , [37] . In contrast, the vast majority of our previous work on Fe/N/C-catalysts involved the use of carbon black supports [23] , [24] , [37] , [38] , [39] . The synthesis method for the Fe/N/C-catalysts in this work consists of preparing a catalyst precursor from iron(II) acetate (FeAc), 1,10-phenanthroline (Phen) and ZIF-8 (Z8); mixing them using low-energy ballmilling; and then performing Pyrolysis #1 in argon at 1,050 °C and, optionally, Pyrolysis #2 in ammonia at 950 °C. Although MOFs have been used in creative ways that may impact PEMFC development, such as gas capture [40] , gas separation and purification [41] , hydrogen storage [36] , [42] , anhydrous proton conduction [43] and the synthesis of highly microporous carbons by thermal decomposition [44] , to our knowledge, only two publications are available in the literature that report the use of MOFs to synthesize ORR catalysts [45] , [46] . However, the catalysts in the latter works showed low activity and power density. We report a Fe/Phen/Z8-derived catalyst with a volumetric activity of 230A cm −3 at 0.8V iR-free , the highest reported to date for non-PGM-based ORR catalysts in PEMFCs. A membrane electrode assembly (MEA) using the latter at the cathode and tested in H 2 -O 2 produced a peak power density of 0.91 W cm −2 and a power density of 0.75 W cm −2 at 0.6 V, the latter comparable with that of a state-of-the-art platinum-based cathode having a loading of 0.3 mg Pt cm −2 . 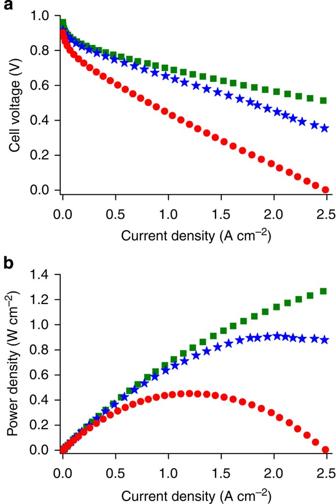Figure 1: Polarization and power density curves of MEAs with Fe-based and Pt-based cathodes. (a) Polarization curves for MEAs comprising a cathode made with 1/20/80-Z8-1050 °C-15 min, the most active Fe/Phen/Z8-derived catalyst in this work (blue stars) and 1/50/50-BP-1050 °C-60 min, our previous most active iron-based catalyst from Lefèvreet al.24(red circles). For comparison, the polarization curve of an MEA made with a state-of-the-art Pt-based cathode with a loading of 0.3 mgPtcm−2(green squares) supplied by an industry leader is also shown. (b) Power density curves corresponding to polarization curves shown ina. For the two MEAs made with iron-based cathodes, the catalyst loading was 3.9 mg cm−2. For all MEAs, NRE 211 membranes were used. Power density of the best Fe-based catalyst in this work The polarization and power density curves of an MEA comprising a cathode made with the best catalyst in this work (blue stars), derived from FeAc/Phen/Z8, and identified as 1/20/80-Z8-1050 °C-15 min, along with that of an MEA comprising a cathode made with our previous most active iron-based catalyst [24] (red circles), identified as 1/50/50-BP-1050 °C-60 min are shown in Figure 1 . The nomenclature used here to identify the Fe/N/C-catalysts is as follows: A/B/C-L-X-Y, where A is the nominal weight percentage of Fe in the catalyst precursor, B/C is the mass ratio of Phen to the microporous host. L is the label for the microporous host (Z8 for ZIF-8 and BP for Black Pearls 2000), X is the temperature of Pyrolysis #1 in argon with a fixed duration of 1 h, and Y is the duration of Pyrolysis #2 in NH 3 , the latter always performed at a temperature of 950 °C. For simplicity, Y =0 min is omitted for all catalysts having undergone Pyrolysis #1 only. A detailed description of the catalyst synthesis is available in the Methods section. Figure 1: Polarization and power density curves of MEAs with Fe-based and Pt-based cathodes. ( a ) Polarization curves for MEAs comprising a cathode made with 1/20/80-Z8-1050 °C-15 min, the most active Fe/Phen/Z8-derived catalyst in this work (blue stars) and 1/50/50-BP-1050 °C-60 min, our previous most active iron-based catalyst from Lefèvre et al . [24] (red circles). For comparison, the polarization curve of an MEA made with a state-of-the-art Pt-based cathode with a loading of 0.3 mg Pt cm −2 (green squares) supplied by an industry leader is also shown. ( b ) Power density curves corresponding to polarization curves shown in a . For the two MEAs made with iron-based cathodes, the catalyst loading was 3.9 mg cm −2 . For all MEAs, NRE 211 membranes were used. Full size image At 0.6 V, the cathode made with 1/20/80-Z8-1050 °C-15 min exhibits an increase in power density by a factor of 2.3 compared with the cathode made with 1/50/50-BP-1050 °C-60 min (0.75 versus 0.32 W cm −2 ). The peak power density for 1/20/80-Z8-1050 °C-15 min is 0.91 W cm −2 compared with 0.45 W cm −2 for 1/50/50-BP-1050 °C-60 min ( Fig. 1b ). This increase in power density, to a level much closer to that of Pt-based cathodes, was achieved despite the thickness of this Fe-based cathode (90–120 μm for 3.9 mg cm −2 loading) being greater by a factor of about 6–12 compared with that of typical state-of-the-art Pt-based cathodes (10–15 μm). Achieving high power density despite this drawback, therefore, emphasizes the enhanced mass-transport properties of this Fe/Phen/Z8-derived catalyst. Also shown in Figure 1 is a state-of-the-art Pt-based cathode having a loading of 0.3 mg Pt cm −2 (green squares). The power performance of 1/20/80-Z8-1050 °C-15 min is very close to that of this state-of-the-art Pt-based cathode. The total (cathode+anode) platinum group metal (PGM) loading for the latter MEA, after adding the platinum loading of the state-of-the-art anode, was 0.35 mg cm −2 . This total loading does not yet meet the US department of energy (DOE)'s obsolescent 2010 target of 0.3 mg cm −2 (ref. 30 ) and is still almost a factor 3 higher than the recently revised 2015 target of ≤0.125 mg PGM cm −2 (ref. 47 ). Ballmilling effect on properties of the catalyst precursor Before carrying out the optimization steps necessary to achieve the optimal power performance, X-ray diffraction (XRD), BET surface area measurement and transmission electron microscopy (TEM) were conducted to investigate the pristine Z8, ballmilled Z8 and the catalyst precursor (a ball milled mixture with 1/20/80 mass ratio of Fe/Phen/Z8). Pristine Z8 is a highly crystalline material with a BET surface area of upto 1,800 m 2 g −1 . The as-received form of the latter consists of well-formed individual crystallites. 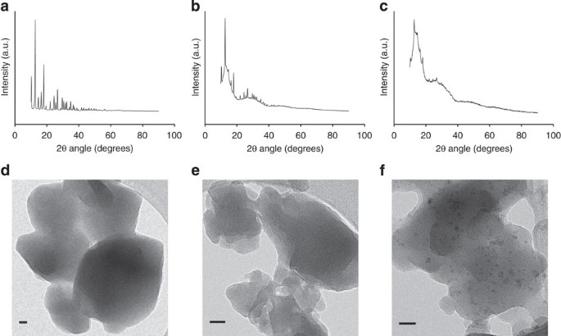Figure 2: XRD and TEM of pristine Z8, ballmilled Z8 and ballmilled catalyst precursor. (a) X-ray diffraction (XRD) of as-received pristine Z8. (b) XRD of ballmilled Z8. (c) XRD of the catalyst precursor for 1/20/80-Fe/Phen/Z8. (d) TEM image of as-received pristine Z8 (scale bar, 20 nm). (e) TEM image of ballmilled Z8 (scale bar, 20 nm). (f) TEM image of the catalyst precursor for 1/20/80-Fe/Phen/Z8 (scale bar, 20 nm). The dark spots observed infwere identified as iron-containing particles using parallel electron energy loss spectroscopy. An XRD and TEM image of pristine Z8 is shown in Figure 2a,d for reference. Figure 2: XRD and TEM of pristine Z8, ballmilled Z8 and ballmilled catalyst precursor. ( a ) X-ray diffraction (XRD) of as-received pristine Z8. ( b ) XRD of ballmilled Z8. ( c ) XRD of the catalyst precursor for 1/20/80-Fe/Phen/Z8. ( d ) TEM image of as-received pristine Z8 (scale bar, 20 nm). ( e ) TEM image of ballmilled Z8 (scale bar, 20 nm). ( f ) TEM image of the catalyst precursor for 1/20/80-Fe/Phen/Z8 (scale bar, 20 nm). The dark spots observed in f were identified as iron-containing particles using parallel electron energy loss spectroscopy. Full size image A notable change in the BET surface area (474 m 2 g −1 ), XRD ( Fig. 2b ), and a discernable change in TEM image ( Fig. 2e ) is observed after pristine Z8 undergoes 3 h of ballmilling. The sharp drop in BET surface area, combined with broadened XRD diffraction peaks ( Fig. 2b ), indicates that the majority of ballmilled Z8 has become a significantly more amorphous material compared with pristine Z8. Owing to the relatively low elastic modulus and hardness of pristine Z8, which can be attributed to their flexible Zn-Imidazolate-Zn linkages [48] , it is known that even manual packing of Z8 produces a marked reduction in crystallinity and structural order [49] , let alone planetary ballmilling for 3 h. Pristine Z8 is therefore highly compressible with an irreversible pressure-induced amorphization at extremely low pressures (in this work, pressure was applied to Z8 by ballmilling). It was also reported that pressure-treated and amorphized Z8 still exhibits nanoporosity and retains some structural order [49] . The same conclusions were reached in this work based on the characterization of ballmilled Z8, which has a BET surface area of 474 m 2 g −1 and some visible diffraction peaks ( Fig. 2b ). Ballmilling of the Fe/Phen/Z8 catalyst precursor resulted in a yet lower BET surface area of only 40 m 2 g −1 compared with that of ballmilled Z8 alone (474 m 2 g −1 ), whereas the XRD diffractograms of both materials are similar ( Fig. 2b,c ). It is believed that the dispersion of Fe/Phen mixture over ballmilled Z8 particles ( Fig 2f ) blocks access to a significant fraction of their internal microporous surface area. This explains why the BET surface area of ballmilled Fe/Phen/Z8 catalyst precursor is only 40 m 2 g −1 , which is much lower than that of ballmilled Z8 alone. Catalytic activity optimization of Fe/Phen/Z8-based catalyst Following the preliminary experiments described above, we optimized the Fe/Phen/Z8-derived catalyst by investigating the effect of the following parameters on the catalytic activity: the temperature of Pyrolysis #1 in Ar for 60 min (X in the catalyst nomenclature: A/B/C-L-X-Y); the time of Pyrolysis #2 in NH 3 at 950 °C (Y); the mass ratio of Phen to microporous host in the catalyst precursor (B/C); and the Fe content in the catalyst precursor (A in the catalyst nomenclature). From our investigation on the effect of the temperature of Pyrolysis #1 in Ar with a 1/20/80 mass ratio Fe/Phen/Z8 catalyst precursor, it was found that pyrolysis of the ballmilled catalyst precursor in Ar at 400 °C resulted in the recrystallization of the amorphized Z8 from ballmilling. Consequently, the Z8 particles in the catalyst precursor regained, in large part, their original crystalline structure as evidenced by the almost identical XRDs for 1/20/80-Z8-400 °C ( Supplementary Fig. S1 ) and pristine Z8 ( Fig. 2a ). However, the microscopic morphology of 1/20/80-Z8-400 °C ( Supplementary Fig. S1 ) remained very similar to that of the ballmilled catalyst precursor ( Fig. 2f ) because ballmilled Z8 is still chemically stable at 400 °C. Based on thermogravimetric analysis (TGA), decomposition begins near or above 500 °C ( Supplementary Fig. S2 ). From TGA, we also observe that the weight loss experienced by the ballmilled catalyst precursor during pyrolysis in Ar while ramping to 400 °C was about 20 wt%, mostly ascribed to the gasification of phenanthroline. A pyrolysis at 700, 850 or 1,050 °C in Ar transforms the Fe/Phen/Z8 precursor into a disordered carbonaceous material (from XRD) with alveolar structures as observed from TEM ( Supplementary Fig. S1 ). Decomposition of Z8 is also confirmed by the increased mass loss and decreased N and Zn content with increasing temperature ( Supplementary Fig. S1 ; Table 1 ). The transformation of the precursor into a nitrogen-containing microporous catalyst is also evidenced from changes in nitrogen coordination observed from X-ray photoelectron spectroscopy (XPS) N1s narrow scans ( Supplementary Fig. S1 ) and increased micropore surface area ( Table 1 ) with increasing temperature, for T ≥700 °C. Table 1 Physical and chemical characterization of selected catalysts. Full size table For catalysts pyrolyzed in Ar the catalytic activity increased with increasing temperature, reaching a reasonably high value of 254 A g −1 at 0.8 V iR-free (based on the extrapolation of the Tafel slope) for 1/20/80-Z8-1050 °C ( Supplementary Fig. S1 ). However, at 0.6 V, the measured specific current (expressed in A g −1 of cathode catalyst) of 1/20/80-Z8-1050 °C was only 100 A g −1 with a loading of 1 mg cm −2 , corresponding to a current density of 0.1 A cm −2 . Next, these catalysts pyrolyzed in Ar at various temperatures underwent Pyrolysis #2 in NH 3 at 950 °C, for different times. The highest ORR-activity was obtained for the catalyst having undergone Pyrolysis #1 in Ar at 1,050 °C for 1 h, followed by pyrolysis #2 in NH 3 at 950 °C for 15 min (1/20/80-Z8-1050 °C-15 min). The activity of the latter catalyst was 1,120 A g −1 at 0.8 V iR-free ( Supplementary Fig. S3 ), compared with only 254 A g −1 for 1/20/80-Z8-1050 °C ( Supplementary Fig. S1 ). The increase in catalytic activity by a factor of 4.4 following Pyrolysis #2 is explained by the general increase in microporous surface area ( Supplementary Fig. S4 ) and N content ( Table 1 ). We also investigated the effect of the Phen content (from 0 to 75 wt%) in the catalyst precursor on the catalytic activity at 0.8V iR-free . With the exception of 0 and 75 wt%, the catalytic activity was relatively independent of Phen content. On the other hand, the power density at 0.6 V was much more sensitive to Phen content, attaining a maximum for 20 wt% Phen ( Supplementary Fig. S5 ). Next, using the optimum 20 wt% for the Phen content, we found that the catalytic activity at 0.8 V iR-free of catalysts made with 0.5 and 1.5 wt%Fe in their respective catalyst precursors was lower than those made with 1 wt% Fe and their power densities at 0.6 V were about 10% lower as well. It should be noted that when iron was omitted from the catalyst precursor, the catalytic activity was three orders of magnitude lower, emphasizing the importance of iron for high activity. Hence, after all optimization steps, the most active catalyst made in this work was 1/20/80-Z8-1050 °C-15 min, with a catalytic activity of 1,120 A g −1 at 0.8 V iR-free (inserts in Supplementary Fig. S3 or S5 ), an increase by a factor of about 2.6 compared with our previous best result of 429 A g −1 (ref. 24 ). Determination of the volumetric activity at 0.8 V iR-free Whereas A g −1 (mass activity) is an acceptable unit for comparing the catalytic activity of non-precious metal catalysts, the preferred units by the US DOE is A cm −3 cathode (volumetric activity) [30] . In addition, the US DOE has defined targets of volumetric activity for non-PGM catalysts for ORR at 0.8 V iR-free under the following reference conditions: 80 °C fuel cell temperature, 1 bar absolute pressure for H 2 and O 2 (excluding water vapour pressure) and 100% relative humidity [30] . To report volumetric activity under US DOE reference conditions, we corrected our mass activity values measured at 0.8 V iR-free and 1.5 bar H 2 and O 2 to 1 bar and converted A g −1 catalyst into A cm −3 cathode , as done in our previous work (see supporting material of ref. 24 ). However, since the catalyst in this work is different from that in ref. 24 , we experimentally determined its corresponding average effective cathode density, which was found to be 0.37 g catalyst cm −3 cathode . The value of ρ eff used in ref. 24 was 0.4 g catalyst cm −3 cathode . 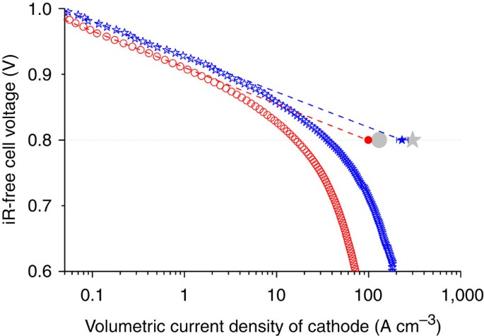Figure 3: Tafel plots for determination of volumetric activity of cathode. Plots presenting iR-free cell voltage versus the log of volumetric current density of cathode for MEAs comprising a cathode made with 1/20/80-Z8-1050 °C-15 min, the most active iron-based catalyst in this work (hollow blue stars) and 1/50/50-BP-1050 °C-60 min, our previous most active iron-based catalyst (hollow red circles)24. The original data to construct these Tafel plots were obtained from H2-O2fuel cell tests with O2and H2absolute pressures of 1.5 bar and converted to US DOE reference conditions, that is, 1 bar absolute pressure for H2and O2. For both MEAs, the cathode catalyst loading was ca. 1 mg cm−2and N117 membranes were used. The current range along the linear region of the Tafel plot used for the extrapolation of the volumetric activity of 1/20/80-Z8-1050 °C-15 min to 0.8 V (dashed blue line), resulting in a value of 230 A cm−3(solid blue star), was 0.05 to 3 A cm−3. The average effective cathode density used for the latter to convert from specific activity (A g−1) to volumetric activity (A cm−3) was 0.37 gcatalystcm−3cathode. The cathode thickness used to determine effective cathode density was measured using SEM of cross-sections of membrane electrode assemblies. Based on the minimum and maximum cathode thicknesses as measured by SEM, the minimum and maximum effective cathode densities were found to be 0.32 and 0.43 gcatalystcm−3cathode, respectively. The error bar attached to the solid blue star represents the minimum and maximum volumetric activity of 1/20/80-Z8-1050 °C-15 min based on the latter. The volumetric activity of 1/50/50-BP-1050 °C-60 min, our previous most active iron-based catalyst, was 99 A cm−3(solid red circle). Also shown for reference are the US DOE volumetric activity targets at 0.8 ViR-freefor non-platinum-group-metal-based oxygen reduction catalysts for the year 2010 (130 A cm−3, solid grey circle) and the year 2015 (300 A cm−3, solid grey star). Figure 3 shows the Tafel plots of 1/20/80-Z8-1050 °C-15 min (hollow blue stars) and 1/50/50-BP-1050 °C-60 min (hollow red circles), as well as the 2010 (large grey circle) and 2015 (large grey star) US DOE volumetric activity targets for non-PGM-based catalysts for ORR in PEMFC. The volumetric activity at 0.8 V iR-free cell voltage is the intersection of the extrapolated Tafel slope (dashed lines) with the 0.8 V iR-free axis. We observe an increase in volumetric activity at 0.8 V iR-free for 1/20/80-Z8-1050 °C-15 min (230 A cm −3 ) by a factor of ca. 2.3 compared with 1/50/50-BP-1050 °C-60 min (99 A cm −3 ) [24] . Figure 3: Tafel plots for determination of volumetric activity of cathode. Plots presenting iR-free cell voltage versus the log of volumetric current density of cathode for MEAs comprising a cathode made with 1/20/80-Z8-1050 °C-15 min, the most active iron-based catalyst in this work (hollow blue stars) and 1/50/50-BP-1050 °C-60 min, our previous most active iron-based catalyst (hollow red circles) [24] . The original data to construct these Tafel plots were obtained from H 2 -O 2 fuel cell tests with O 2 and H 2 absolute pressures of 1.5 bar and converted to US DOE reference conditions, that is, 1 bar absolute pressure for H 2 and O 2 . For both MEAs, the cathode catalyst loading was ca. 1 mg cm −2 and N117 membranes were used. The current range along the linear region of the Tafel plot used for the extrapolation of the volumetric activity of 1/20/80-Z8-1050 °C-15 min to 0.8 V (dashed blue line), resulting in a value of 230 A cm −3 (solid blue star), was 0.05 to 3 A cm −3 . The average effective cathode density used for the latter to convert from specific activity (A g −1 ) to volumetric activity (A cm −3 ) was 0.37 g catalyst cm −3 cathode . The cathode thickness used to determine effective cathode density was measured using SEM of cross-sections of membrane electrode assemblies. Based on the minimum and maximum cathode thicknesses as measured by SEM, the minimum and maximum effective cathode densities were found to be 0.32 and 0.43 g catalyst cm −3 cathode , respectively. The error bar attached to the solid blue star represents the minimum and maximum volumetric activity of 1/20/80-Z8-1050 °C-15 min based on the latter. The volumetric activity of 1/50/50-BP-1050 °C-60 min, our previous most active iron-based catalyst, was 99 A cm −3 (solid red circle). Also shown for reference are the US DOE volumetric activity targets at 0.8 V iR-free for non-platinum-group-metal-based oxygen reduction catalysts for the year 2010 (130 A cm −3 , solid grey circle) and the year 2015 (300 A cm −3 , solid grey star). Full size image We then maximized the power density at 0.6 V by choosing a thinner polymer electrolyte membrane (Nafion NRE-211 membrane, 25 μm thick) than that used for the activity measurements (N117, 175 μm thick) and by optimizing the cathode catalyst loading ( Supplementary Fig. S6 ). The highest current density at 0.6 V (1.25 A cm −2 ) under H 2 /O 2 (1.5 bar absolute pressure) was obtained with a cathode loading of 3.9 mg cm −2 ( Supplementary Fig. S6 ). The latter polarization curve and its corresponding power density curve are those shown in Figure 1 . According to the Tafel law, the increase by a factor of ca. 2.3 in ORR volumetric activity of 1/20/80-Z8-1050 °C-15 min can only contribute at most an improvement of ca. 20 mV at any current density compared with 1/50/50-BP-1050 °C-60 min. However, the voltage gap between the polarization curves of 1/20/80-Z8-1050 °C-15 min and 1/50/50-BP-1050 °C-60 min observed in Figure 1a is always greater than 20 mV and increases with increasing current density to a maximum of 350 mV. Therefore, the vast majority of the over-twofold increase in current density at 0.6 V ( Fig. 1a ) can only be explained by improved mass-transport properties of the catalyst or the catalyst–ionomer layer structure. Improved mass-transport properties intrinsic to the catalyst should be reflected by a change in one or several of its characteristics. Compared with 1/50/50-BP-1050 °C-60 min, 1/20/80-Z8-1050 °C-15 min particularly shows increased BET, micropore and mesopore surface areas as well as nitrogen and iron contents ( Table 1 ). Although the latter characteristics may contribute to increased catalytic activity, they are expected to have little or no effect on mass-transport properties. More compelling evidence for the improvement in mass-transport properties is best highlighted by electronic microscopies. 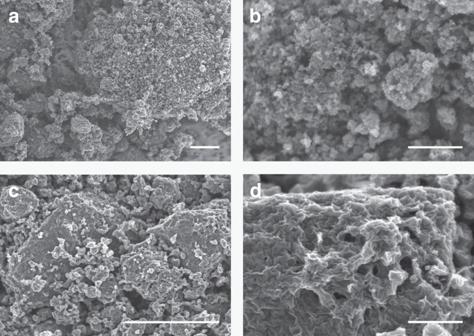Figure 4: Morphology and structure comparison of Fe-based catalysts from SEM. (a) Lower magnification SEM image of 1/50/50-BP-1050 °C-60 min, our previous most active iron-based catalyst from Lefèvreet al.24(scale bar, 4 μm). (b) Higher magnification SEM image of 1/50/50-BP-1050 °C-60 min (scale bar, 500 nm). (c) Lower magnification SEM image of 1/20/80-Z8-1050 °C-15 min, the most active iron-based catalyst in this work (scale bar, 4 μm). (d) Higher magnification SEM image of 1/20/80-Z8-1050 °C-15 min (scale bar, 500 nm). Figure 4a,d show scanning electron microscopy (SEM) images for both catalysts: 1/50/50-BP-1050 °C-60 min and 1/20/80-Z8-1050 °C-15 min. Whereas the surface topology of the catalyst made with BP ( Fig. 4a,b ) shows large particles resulting from the aggregation of smaller particles (20–40 nm), SEM micrographs of the catalyst made with Z8 ( Fig. 4c,d ) show many particles with more defined geometries, similar to the original Z8 crystallites. Furthermore, a close-up of the latter particles ( Fig. 4d ) shows that they contain numerous pores of about 50 nm diameter through which the circulation of oxygen and water is certainly facilitated. 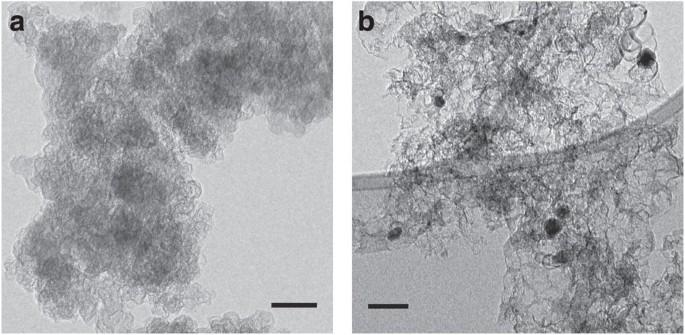Figure 5: Morphology and structure comparison of Fe-based catalysts from TEM. (a) TEM image of 1/50/50-BP-1050 °C-60 min, our previous most active iron-based catalyst from Lefèvreet al.24(scale bar, 50 nm). (b) TEM image of 1/20/80-Z8-1050 °C-15 min, the most active iron-based catalyst in this work (scale bar, 50 nm). From TEM images, we also observe important differences in the carbon structure, as shown in Figure 5 . Whereas the TEM image of 1/50/50-BP-1050 °C-60 min (see Fig. 5a ) shows a dense agglomerated particulate structure consisting of 20–40 nm size particles, that of 1/20/80-Z8-1050 °C-15 min ( Fig. 5b ) shows a seemingly interconnected hollower structure, having typical wall thicknesses of less than 10 nm. Therefore, it is clear that the diffusion of ORR-related species towards and away from the catalytic sites located in the micropores of the hollower-structured 1/20/80-Z8-1050 °C-15 min is facilitated compared with that in the micropores of the denser particulate structure of 1/50/50-BP-1050 °C-60 min. Whereas other research groups such as those of Bogdanoff [50] , [51] , Atanassov [52] and Dahn [53] , [54] have synthesized M/N/C-catalysts using a foaming agent or mesoporous silica templates to control the pore structure of the final catalysts, instead of resorting to carbon blacks or charcoals, none of these approaches led to a breakthrough in power density. Moreover, the use of MOFs per se in the synthesis of non-PGM-based catalysts did not yield better performing ORR catalysts either [45] , [46] . In the latter work the MOF used was a Co-based ZIF, unlike the Zn-based ZIF used here. A key difference in the catalyst syntheses is that Zn mostly escapes during pyrolysis, while Co does not. This raises the questions as to whether the departure of Zn during synthesis has an active role in the formation of the pore structures observed in this work. Figure 4: Morphology and structure comparison of Fe-based catalysts from SEM. ( a ) Lower magnification SEM image of 1/50/50-BP-1050 °C-60 min, our previous most active iron-based catalyst from Lefèvre et al . [24] (scale bar, 4 μm). ( b ) Higher magnification SEM image of 1/50/50-BP-1050 °C-60 min (scale bar, 500 nm). ( c ) Lower magnification SEM image of 1/20/80-Z8-1050 °C-15 min, the most active iron-based catalyst in this work (scale bar, 4 μm). ( d ) Higher magnification SEM image of 1/20/80-Z8-1050 °C-15 min (scale bar, 500 nm). Full size image Figure 5: Morphology and structure comparison of Fe-based catalysts from TEM. ( a ) TEM image of 1/50/50-BP-1050 °C-60 min, our previous most active iron-based catalyst from Lefèvre et al . [24] (scale bar, 50 nm). ( b ) TEM image of 1/20/80-Z8-1050 °C-15 min, the most active iron-based catalyst in this work (scale bar, 50 nm). Full size image It should be noted that the Zn content in selected catalysts, as measured using neutron activation analysis (NAA), a bulk analysis technique, and as reported in Table 1 , was 5.94 at% after pyrolysis of the ballmilled catalyst precursor in Ar at 400 °C, 6.71 at% after pyrolysis in Ar at 700 °C, but decreased thereafter when pyrolyzed at higher temperatures, reaching only 0.06 wt% after pyrolysis in Ar at 1,050 °C and finally only 0.01 wt% following the subsequent Pyrolysis #2 in NH 3 at 950 °C. Here Zn content progressively decreases from the catalyst with increasing pyrolysis temperature in Ar, whereas the Fe content, also measured using NAA, increases. On the basis of the experimental data, we propose the following explanation, which remains hypothetical and will require further experiments to confirm. According to the TGA shown in Supplementary Figure S2 , Z8 particles in the ballmilled Fe/Phen/Z8 catalyst precursor withstand thermal decomposition upto about 500 °C above which the Zn II -Imidazolate-Zn II linkages start to decompose releasing CN fragments from the imidazolate linker. The latter fragments may react with Zn II to form Zn(CN) 2 , a solid that thermally decomposes above 800 °C. Thus, most of the initial Zn content in the catalyst precursor is expected to be present in the catalyst even after a pyrolysis at 700 °C in Ar. Consequently, Because the mass loss experienced at 700 °C (29.8%) is greater than at 400 °C (12.5%), the Zn content (in at%) is expected to be greater as well ( Table 1 ). At 850 °C, Zn(CN) 2 is well above its decomposition temperature and produces Zn and CN fragments, likely as hydrogen cyanide or perhaps cyanogen. The latter volatile decomposition products escape the heat-treated catalyst following the same route as other volatile organic material produced at lower temperatures. The advantage in working with a Zn-imidazolate MOF is that Zn, which is likely reduced to a metallic phase after decomposition of Zn(CN) 2 at temperatures above ca. 800 °C , develops a considerable vapour pressure at 850 °C (nearly 50 kPa) [55] and has a boiling point of only 907 °C. Zn vapour will therefore escape through existing routes previously formed by the release of volatile organic material during carbonization and is therefore not responsible for pore formation in the catalyst. Because the vapour pressure of Zn at 1,050 °C is greater than at 850 °C, it is expected that more Zn will escape the catalyst on pyrolysis at 1,050 °C ( Table 1 ). The subsequent Pyrolysis #2 at 950 °C in NH 3 further decreases Zn content because it allows more time for Zn vapours to escape at a temperature above its boiling point. The latter pyrolysis also etches the disordered carbon in the catalyst to produce further mass loss and consequently produces extra microporosity, possibly allowing otherwise trapped Zn to escape as well. As the iron in the catalyst precursor is unlikely to escape the catalyst during pyrolysis at temperatures ≤1,050 °C, the iron content in the catalyst is expected to increase with increasing mass loss ( Table 1 ). Ultimately, replacement of Pt-based cathode catalysts with non-PGM-based ones will require both high power density and durability. Hundred-hour stability tests at 0.5 V were performed on 1/20/80-Z8-1050 °C-15 min and 1/20/80-Z8-1050 °C, both in H 2 -O 2 and H 2 -Air ( Fig. 6a,b ). The stability tests in both cases show that the current density with 1/20/80-Z8-1050 °C-15 min decays faster than with 1/20/80-Z8-1050 °C. The best stability was obtained with 1/20/80-Z8-1050 °C in H 2 /Air, with a drop in current density of only 15% at 0.5 V over 100 h. Hence, major improvement in durability is still required, especially for the most active catalyst obtained after Pyrolysis #2 in NH 3 . The power performance of 1/20/80-Z8-1050 °C is, however, comparable with that of most durable M/N/C-catalysts reported to date [26] , [27] , [56] . 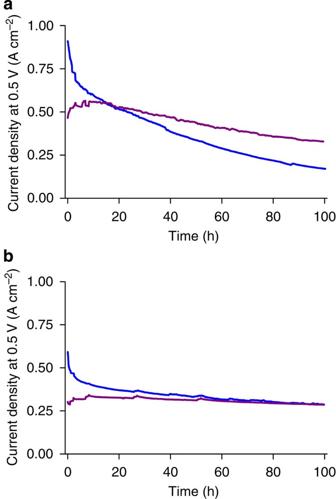Figure 6: 100-h H2-O2and H2-Air current stability curves for MEAs with Fe-based cathodes. (a) Current stability curves at 0.5 V cell voltage performed in H2-O2for a MEA comprising a cathode made with 1/20/80-Z8-1050 °C-15 min, the most active iron-based catalyst in this work (blue curve) and a MEA comprising a cathode made with 1/20/80-Z8-1050 °C, prepared using 20/80 Phen/Z8 mass ratio and 1 wt% Fe in the catalyst precursor and undergoing only Pyrolysis # 1 in Ar at 1,050 °C for 60 min (purple curve). (b) Current stability curves at 0.5 V cell voltage performed in H2-Air for MEAs comprising cathodes made with 1/20/80-Z8-1050 °C-15 min (blue curve) and 1/20/80-Z8-1050 °C (purple curve). The cathode catalyst loading used was ca. 3.9 mg cm−2, the anode GDE was 0.5 mgPtcm−2, and the membrane was N117. The back pressures for all gases in all tests was 2 bar gauge. Figure 6: 100-h H 2 -O 2 and H 2 -Air current stability curves for MEAs with Fe-based cathodes. ( a ) Current stability curves at 0.5 V cell voltage performed in H 2 -O 2 for a MEA comprising a cathode made with 1/20/80-Z8-1050 °C-15 min, the most active iron-based catalyst in this work (blue curve) and a MEA comprising a cathode made with 1/20/80-Z8-1050 °C, prepared using 20/80 Phen/Z8 mass ratio and 1 wt% Fe in the catalyst precursor and undergoing only Pyrolysis # 1 in Ar at 1,050 °C for 60 min (purple curve). ( b ) Current stability curves at 0.5 V cell voltage performed in H 2 -Air for MEAs comprising cathodes made with 1/20/80-Z8-1050 °C-15 min (blue curve) and 1/20/80-Z8-1050 °C (purple curve). The cathode catalyst loading used was ca. 3.9 mg cm −2 , the anode GDE was 0.5 mg Pt cm −2 , and the membrane was N117. The back pressures for all gases in all tests was 2 bar gauge. Full size image In summary, Fe-based catalysts for PEMFCs were prepared from a mixture of a Zn(II) ZIF, 1,10-phenanthroline and ferrous acetate. The mixture was ballmilled, pyrolyzed twice, first in argon at 1,050 °C, then in ammonia at 950 °C. A membrane electrode assembly using the best catalyst in this work at the cathode produced a power density comparable with that of a state-of-the-art platinum-based cathode having a loading of 0.3 mg Pt cm −2 . Its volumetric activity is the highest reported to date for a non-PGM catalyst for oxygen reduction in a PEMFC and is now much closer to the US DOE's 2015 target of ≥300 A cm −3 (ref. 47 ). Based on scanning and TEM images, it is believed that the interconnected alveolar carbon nanostructure of Fe/Phen/Z8-derived catalysts is at the root of the observed enhanced mass-transport properties in the cathodes studied in this work. The unprecedented catalytic activity and power density of these new Fe-based catalysts bolster the prospect of a viable alternative to Pt-based cathode catalysts in PEMFCs. The focus of continued research and development has now turned to improving the durability of these otherwise highly active and now well-performing iron-based catalysts. Catalyst precursor and catalyst preparation The catalysts in this work were prepared using various mass ratios of three components: a microporous host, ZIF-8 (Basolite Z1200, Aldrich, produced by BASF) or Black Pearls 2000 (Cabot); small nitrogen-containing organic molecules, Phen (1,10-Phenanthroline, ≥99%, Aldrich); and an iron salt, FeAc (Iron(II) acetate, 95%, Aldrich). Catalyst precursors (that is, the powder mixtures prepared to be subsequently pyrolyzed) were prepared by first mixing ZIF-8 (Z8), Phen and FeAc in a solution of ethanol and deionized water (1:2 ethanol/H 2 O), then drying the slurry. The dry powder was then placed in a hardened steel vial (ca. 65 cm 3 ) with 20 chrome steel balls of 0.25 inch diameter. Typically, ca. 1 g of powder was ballmilled at once. The ball-to-powder mass ratio was ca. 20:1. The vial was sealed in a nitrogen glove box. Once tightly sealed, the vial was placed in a planetary ballmiller (FRITSCH Pulverisette 7) to undergo 3 h of ballmilling at 400 r.p.m. The resulting dry powder was the catalyst precursor. The catalyst precursor then underwent one or two pyrolyses in either Ar or NH 3 . Precise control on the pyrolysis temperature and duration was achieved through a procedure that is described in detail in Jaouen et al . [31] Preparation of cathode catalyst inks The catalyst inks in this work were prepared using the following formulation (corresponding to an ionomer-to-catalyst ratio of 1.5): 10 mg of catalyst was mixed in a glass vial with 326 μl of Nafion 5 wt% dispersion solution (Aldrich), 163 μl of ethanol and 136 μl of deionized water. The inks were sonicated and agitated in a vortex mixer for a total of 1 h. These catalysts inks were then used to prepare the cathode for fuel cell testing. Preparation of cathodes and anodes For catalytic activity measurements in PEMFC, 71 μl of catalyst ink was deposited for each 1 mg cm −2 of cathode catalyst loading on an uncatalysed round 1.14 cm 2 substrate (a custom made gas diffusion layer consisting of an ElectroChem EC-CC1-060 T Teflon-treated carbon cloth covered on both sides with a microporous layer of ca. 2.3 mg cm −2 of Vulcan XC-72 and an equal mass of Teflon). The anode used for all PEM FC tests performed with iron-based cathode catalysts in this work was a custom made gas diffusion electrode (GDE) consisting of a substrate (same as described above for cathode) with a catalyst layer of 46 wt% platinum on Vulcan XC-72 by Tanaka Kikinzoku with a catalyst loading of 0.5 mg cm −2 and an ionomer-to-carbon ratio of 2. The anode and cathode were then placed in a vacuum oven at ca. 80 °C to dry for 1 h. The mass of catalyst in the cathode was determined by subtracting the mass of the uncatalysed substrate from the dry mass of the catalyst-coated substrate and dividing the remainder by [ionomer-to-catalyst ratio+1]. For the MEAs made with Pt-based cathodes, state-of-the-art anodes having a loading of 0.05 mg Pt cm −2 were used. For?all fuel cell tests in this work, the anode platinum loading was sufficient to ensure that the anode reaction was non-limiting. Anodes for the platinum-based cathode MEAs were supplied by industry. Anodes for iron-based cathode MEAs were prepared in-house as described above. It has been demonstrated that a loading of greater than 0.05 mg Pt cm −2 at the anode has no appreciable effect on the polarization curves [28] , [57] , [58] . Preparation of membrane electrode assemblies MEAs were prepared by hot-pressing round 1.14 cm 2 anode and cathode GDEs against either side of either a Nafion N117 or NRE 211 membrane at ca. 140 °C for 40 s using a load of ca. 500 lb. When preparing MEAs using Nafion NRE211 membranes, the cathodes were first smoothed by pre-pressing the cathode at ca. 140 °C for 40 s using a load of ca. 500 lb. to minimize the risk of puncturing the membrane during MEA hot pressing. Activity and stability fuel cell testing PEM FC tests in this work were performed using MEAs in a single-cell test fuel cell using a GlobeTech GT60 fuel cell test bench and a BioLogic SP-150 Potentiostat with a VMP3B-20 Booster and EC-Lab V9.98. software. Teflon gaskets were used at both the anode and cathode sides. The gasket thicknesses were chosen to achieve ca. 15–25% compression of the gas diffusion+catalyst layers. For activity and performance tests, the fuel cell temperature was 80 °C, the back pressures were set to ca. 1 bar gauge for both anode and cathode sides. Thus, the absolute pressure for both H 2 and O 2 was 1.5 bars (with ca. 0.5 bar partial pressure attributed to water vapour at ca. 80 °C). The flow rates for H 2 and O 2 were ca. 0.3 slpm using fully humidified gases. In the case of the Pt-based cathode MEA, the anode and cathode were fully activated before measuring the polarization curve. First, an electrochemical impedance spectroscopy measurement was performed at open circuit voltage, with frequencies ranging from 50 kHz down to 10 Hz to measure the fuel cell resistance for iR-correction. A polarization curve was then recorded by scanning the cell voltag e from open circuit voltage down to 0 V at a scan rate of 0.5 mV s −1 . H 2 /O 2 and H 2 /air stability measurements using MEAs were performed in a single-cell test fuel cell. The cell voltage was held at 0.5 V for 100 h and the current was recorded. However, polarization curves were measured at various times throughout stability testing, that is, initially, and after 1, 6, 24, 48 and 96 h of operation at 0.5 V. The fuel cell temperature was 80 °C; all gases were at 100% RH; and the back pressure was 2 bar gauge on both sides. All gas flow rates were 0.3 slpm. The fuel cell voltage and back pressures used in this work, that is, 0.5 V and 2 bar gauge, respectively, were specifically chosen to allow an 'apple-to-apple' comparison with stability test results of other non-PGM-based cathode catalysts from published literature. Thermogravimetric analysis TGA was conducted using a Thermogravimetric/Differential Thermal Analyzer (TG/DTA200, Seiko Instrument). All measurements were carried out under nitrogen with a flow rate of 100 ml min -1 . The samples were heated from room temperature to 1000 °C at a ramp rate of 15 °C min -1 . A cylindrical platinum crucible was used for analysing these samples. Before each experiment, to remove impurities, the platinum crucible was heated with a torch until it became red hot (>1100 °C). Physical and chemical characterization Surface area measurement of catalysts was performed with a Quantachrome Instruments Autosorb-1 and with N 2 as the adsorbate. The surface areas were estimated from the BET equation and from the fitting of the N 2 -adsorption isotherms obtained using Autosorb-1 surface area analyser from Quantachrome Instruments, with the Quenched solid density functional theory (slit-pore geometry) available in the AS1WIN software. Micropores are defined as pores having sizes less than or equal to 2 nm, mesopores between 2 and 50 nm, and macropores as greater than 50 nm. Surface atomic ratio of catalysts was measured by XPS using a VG Escalab 200i instrument. The Al Kα line (1486.6 eV) was chosen as the X-ray source. The quantification of the elements was performed using CasaXPS software. Bulk Fe and Zn content was measured by NAA at École Polytechnique de Montréal. Bragg–Brentano XRD was performed with a Bruker D8 diffractometer using Cu Kα radiation. TEM was used to analyse the structure and nanostructure of the catalysts. TEM was also used to qualitatively analyse the local composition of the catalysts (for the carbon structures and the metal particles). For the preparation of the samples, a copper grid partially covered with an amorphous carbon film was dipped into a methanol solution containing the catalyst and was dried. The solution was previously produced by ultrasonically dispersing the catalyst (about 10 mg) into methanol (about 2 ml) for ca. 1 min. For the TEM measurements, a JEOL 2100F microscope was used with an acceleration voltage of 200 kV and a typical current density of 15 pA cm −2 . Images were obtained in bright field. Parallel electron energy loss spectroscopy was also performed for elemental analysis. SEM was used to analyse the structure and morphology of the catalysts and to analyse GDE and MEA cross-sections for cathode thickness measurements. For these measurements, the catalyst powder was directly pressed onto an aluminum tape. For the SEM measurements, a Hitachi S4700 (with a field emission gun) was used at an acceleration voltage of 2 kV. How to cite this article: Proietti, E. et al . Iron-Based Cathode Catalyst with Enhanced Power Density in Polymer Electrolyte Membrane Fuel Cells. Nat. Commun. 2:416 doi: 10.1038/ncomms1427 (2011).